Quantum signatures of a molecular nanomagnet in direct magnetocaloric measurements Geometric spin frustration in low-dimensional materials, such as the two-dimensional kagome or triangular antiferromagnetic nets, can significantly enhance the change of the magnetic entropy and adiabatic temperature following a change in the applied magnetic field, that is, the magnetocaloric effect. In principle, an equivalent outcome should also be observable in certain high-symmetry zero-dimensional, that is, molecular, structures with frustrated topologies. Here we report experimental realization of this in a heptametallic gadolinium molecule. Adiabatic demagnetization experiments reach ~200 mK, the first sub-Kelvin cooling with any molecular nanomagnet, and reveal isentropes (the constant entropy paths followed in the temperature-field plane) with a rich structure. The latter is shown to be a direct manifestation of the trigonal antiferromagnetic net structure, allowing study of frustration-enhanced magnetocaloric effects in a finite system. Sub-Kelvin temperatures can be achieved via adiabatic demagnetization of paramagnetic salts [1] , [2] . The underlying physics is the magnetocaloric effect (MCE) that can be evaluated by considering the adiabatic temperature change, which is when the system is driven on a constant entropy ( S ) curve (an isentrope): where C is the heat capacity, T is the temperature and B is the applied magnetic field. For a paramagnet, the isentropes are straight lines in a T – B plane that run through the origin. Interacting spin systems can show a much richer response to magnetic fields and thus very different isentropes. Importantly, the cooling rate can massively outperform those of paramagnets in certain regions of the T – B plane [3] . The simplest illustration is an antiferromagnetically coupled dimer of s =1/2 spin ( Fig. 1 ) where extremes in the cooling rates (even changing sign) are found at the field-induced level crossing between singlet and triplet because the density of states (and hence the low-temperature entropy) peaks at this field. 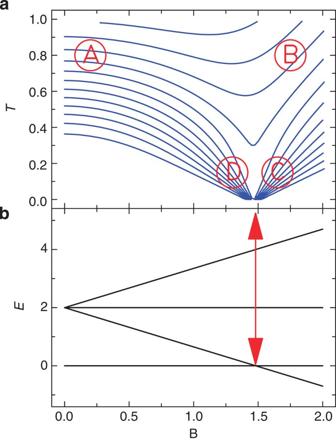Figure 1: Theoretical isentropes for an antiferromagnetically coupled dimer ofs=1/2 spins. (a) Calculated isentropes in the temperature (T)–applied magnetic field (B) plane for the dimer with the Zeeman diagram inb. The two lowest-energy Zeeman levels cross at a field that depends on the magnitude of the exchange coupling, giving a maximum in the density of states. Simple paramagnets have linear isentropes, always giving a decrease inTasBis decreased. While the cooling rate for the antiferromagnetically coupled dimer is similar in the highT–Bregion (B), in other regions it can be reduced (A), drastically enhanced (C) or even have the opposite sign (D, that is, heating occurs on decreasing the field). In an adiabatic process (a process of constant entropy), the system runs along its present isentrope. The extreme behaviour at (C) and (D) is due to the level crossing and the consequent rapid changes in entropy. Figure 1: Theoretical isentropes for an antiferromagnetically coupled dimer of s =1/2 spins. ( a ) Calculated isentropes in the temperature ( T )–applied magnetic field ( B ) plane for the dimer with the Zeeman diagram in b . The two lowest-energy Zeeman levels cross at a field that depends on the magnitude of the exchange coupling, giving a maximum in the density of states. Simple paramagnets have linear isentropes, always giving a decrease in T as B is decreased. While the cooling rate for the antiferromagnetically coupled dimer is similar in the high T – B region (B), in other regions it can be reduced (A), drastically enhanced (C) or even have the opposite sign (D, that is, heating occurs on decreasing the field). In an adiabatic process (a process of constant entropy), the system runs along its present isentrope. The extreme behaviour at (C) and (D) is due to the level crossing and the consequent rapid changes in entropy. Full size image Such a crossing belongs to the broader class of quantum phase transitions where the ground-state characteristics of a system change (for example, non-magnetic to magnetic, or from gapped to gapless) as a function of an external parameter such as magnetic field, pressure or doping [4] . For MCE, the drastic changes in entropy across a field-induced quantum critical point can give very efficient low-temperature magnetic cooling as recently demonstrated experimentally for a one-dimensional (1D) antiferromagnetic (AF) s =1/2 chain [3] . Geometric spin frustration can also give rise to regions of high density of states (and zero-temperature entropy), hence very high cooling rates should also be achievable, for example, when sweeping across the saturation field in such materials. The combination of these features in low-dimensional frustrated magnetic materials, for example, the famous 2D kagome or triangular AF lattices or the 1D saw-tooth AF chain [5] , [6] , [7] , [8] , [9] , makes them attractive targets for enhanced MCE and low-temperature refrigeration. In fact, such effects should be also observable in certain 0D systems, that is, molecular clusters of spins in frustrated geometries [10] , [11] , [12] , [13] . These are a subset of the broader class of molecules known as molecular nanomagnets. The molecular cluster [Gd 7 (OH) 6 (thmeH 2 ) 5 (thmeH)(tpa) 6 (MeCN) 2 ](NO 3 ) 2 (‘Gd 7 ’; H 3 thme=tris(hydroxymethyl)ethane; Htpa=triphenylacetic acid) consists of a planar centred hexagon of weakly AF-coupled Gd(III) ions ( Fig. 2 ; ref. 14 ), each of which has an electronic spin s =7/2. Hence, this topology is a finite ‘cutout’ of the 2D triangular AF lattice ( Fig. 2 ). Here we model all the magnetic observables of Gd 7 , including sub-Kelvin susceptibility and heat capacity data. We then use this model to calculate the isentropes for Gd 7 , revealing detailed structure in the T – B landscape due to the frustration. Finally, we follow these isentropes experimentally by direct measurement of the temperature in applied magnetic field cycles under quasi-adiabatic conditions. The experimental data, reproduced by theoretical modelling, show the characteristics of frustration-enhanced MCE; moreover, we achieve cooling to ~200 mK—the first time sub-Kelvin cooling has been achieved with a molecular nanomagnet. 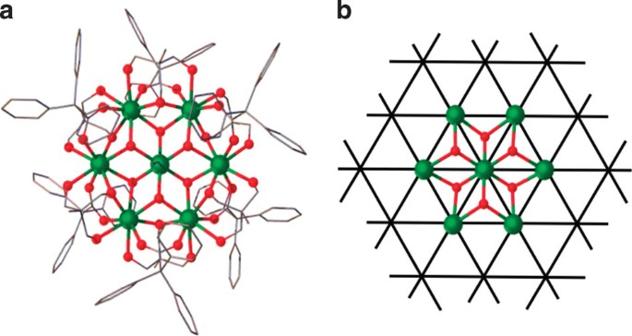Figure 2: Structure of the complex dication of Gd7. Crystal structure (a) and the Gd7(OH)6core mapped onto an ideal triangular net (b), emphasising the relationship of the spin topology with the frustrated triangular AF lattice. Scheme: Gd (green), O (red), N (blue), C (framework), H omitted for clarity. Figure 2: Structure of the complex dication of Gd 7 . Crystal structure ( a ) and the Gd 7 (OH) 6 core mapped onto an ideal triangular net ( b ), emphasising the relationship of the spin topology with the frustrated triangular AF lattice. Scheme: Gd (green), O (red), N (blue), C (framework), H omitted for clarity. Full size image Magnetic properties Low-temperature magnetic data of Gd 7 are summarized in Fig. 3 . The magnetization ( M ) saturates to the maximum possible 49/2 gμ B (where g is the electronic g -factor) per molecule at 2 K, showing that the full magnetic entropy is accessible ( Fig. 3a ). The χT product, where χ is the molar magnetic susceptibility, has the value calculated for non-interacting Gd(III) ions at room temperature (56.2 e.m.u. K mol −1 ) and decreases only slowly on cooling down to ~50 K before decreasing rapidly on further cooling ( Fig. 3b ), denoting a dominant AF interaction. That Gd 7 has a richer physics than a simple paramagnet is manifested in the very-low-temperature susceptibility, which goes through two shallow maxima, at 1–2 K and at 0.2–0.3 K ( Fig. 3b , inset). Above 4 K, the molar heat capacity ( C ) in zero applied field is dominated by lattice phonon modes of the crystal, that is, non-magnetic contributions ( Fig. 3c ). This is confirmed from C ( T ) data on the isostructural and diamagnetic yttrium analogue [Y 7 (OH) 6 (thmeH 2 ) 5 (thmeH)(tpa) 6 (MeCN) 2 ](NO 3 ) 2 (‘Y 7 ’), which overlay those of Gd 7 at higher temperatures. The phonon heat capacity can be described by the Debye model, which simplifies to a C / R = aT 3 dependence ( R is the gas constant), where a =1.35 × 10 −2 K −3 for Gd 7 and Y 7 , at the lowest temperatures. The magnetic contribution to the C ( T ) data for Gd 7 consists of a broad hump that shifts to higher temperature on increasing the applied magnetic field ( Fig. 3c ). 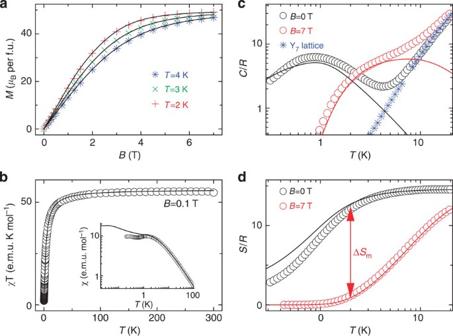Figure 3: Magnetic properties of Gd7. (a) Magnetization (M) as a function of applied magnetic field (B) and temperature (T=2, 3, 4 K), and fits (solid lines) from spin Hamiltonian (2). (b) Molar magnetic susceptibility (χ), in the form ofχTandχ(inset), as a function of temperature, measured in an applied field of 0.1 T, and fits (solid lines). (c) Molar heat capacity (C) of Gd7as a function of temperature atB=0 (black symbols) and 7 T (red), and for its diamagnetic analogue Y7(blue) in nil field giving the lattice (non-magnetic) contribution toC. Solid lines are the calculated magnetic contributions toC(B,T) from Hamiltonian (2). (d) Magnetic molar entropy, as obtained fromC(T) data forB=0 (black) and 7 T (red). Solid lines are the calculated entropies from Hamiltonian (2). Arrows denote the magnetic entropy change, ΔSm(seeSupplementary Fig. 1). The small deviations between theory and experiment seen inχandCat very low temperatures indicate the onset of magnetic dipolar interactions. Figure 3: Magnetic properties of Gd 7 . ( a ) Magnetization ( M ) as a function of applied magnetic field ( B ) and temperature ( T =2, 3, 4 K), and fits (solid lines) from spin Hamiltonian (2). ( b ) Molar magnetic susceptibility ( χ ), in the form of χT and χ (inset), as a function of temperature, measured in an applied field of 0.1 T, and fits (solid lines). ( c ) Molar heat capacity ( C ) of Gd 7 as a function of temperature at B =0 (black symbols) and 7 T (red), and for its diamagnetic analogue Y 7 (blue) in nil field giving the lattice (non-magnetic) contribution to C . Solid lines are the calculated magnetic contributions to C ( B , T ) from Hamiltonian (2). ( d ) Magnetic molar entropy, as obtained from C ( T ) data for B =0 (black) and 7 T (red). Solid lines are the calculated entropies from Hamiltonian (2). Arrows denote the magnetic entropy change, Δ S m (see Supplementary Fig. 1 ). The small deviations between theory and experiment seen in χ and C at very low temperatures indicate the onset of magnetic dipolar interactions. Full size image Magnetic modelling We have modelled all these magnetic data assuming the simple Heisenberg spin Hamiltonian: where J 1 is the exchange interactions between nearest neighbours on the hexagon (spins 1–6), and J 2 is the interactions between each of these spins and the central Gd (spin 7). The huge matrix dimension of 8 7 requires exploiting group theoretical methods [15] , [16] (and the approximate C 6 molecular symmetry) for full matrix diagonalization. We find J 1 =−0.090(5) K, and J 2 =−0.080(5) K with g =2.02 reproduces all the experimental magnetic observables ( Fig. 3 ). Only at the very lowest temperatures, the weak-field susceptibility and zero-field heat capacity show slight deviations between calculated and experimental data. For instance, the calculated susceptibility reproduces the shallow two-peak structure, with the higher-temperature feature agreeing well but the lower temperature one calculated to be at ~0.05 K rather than the experimental 0.2–0.3 K. Most likely, these discrepancies are due to weak magnetic dipolar interactions, which are not incorporated in the theoretical model. Dipolar interactions modify the structure of energy levels and can determine (on the mean-field level) an internal field; both become relevant in proximity of absolute zero and zero applied field. Experimental evaluation of the MCE The MCE can be evaluated indirectly for a given applied field change from the experimental C ( B , T ) (for example, Fig. 3d ) and M ( B,T ) data via Maxwell’s relations [17] : values for Gd 7 derived from these two observables are in very good agreement ( Supplementary Fig. 1 ). Here we have also performed direct experimental measurements of the MCE for continuous field variations, that is, the temperature evolution via magnetization–demagnetization cycles that we perform under controlled quasi-adiabatic conditions, using the set-up and protocols described in Supplementary Note 1 and ref. 18 . Supplementary Fig. 2 displays a representative full magnetic field cycle, and Supplementary Fig. 3 a representative demagnetization process from an initial temperature T 0 =0.50 K and field B 0 =2 T. We show both the raw temperature data and those for an ideal adiabatic process, that is, corrected for unavoidable thermal losses (non-adiabaticity) that have been evaluated independently (see Supplementary Note 1 ). By this method, we experimentally follow isentropes in the T – B plane for different B 0 and T 0 (up to 3 T and 3 K, respectively; Fig. 4 ; Supplementary Fig. 4 ). The general trend is a decrease in T as B is decreased, as expected. There are two important results from these adiabatic demagnetization experiments. First, we achieve temperatures as low as ~ 200 mK. Despite many indirect MCE studies on molecular nanomagnets, this is the first direct experimental demonstration of sub-Kelvin cooling with such a species. Second, in contrast to the straight-line isentropes found for simple paramagnets, a rich structure is observed. 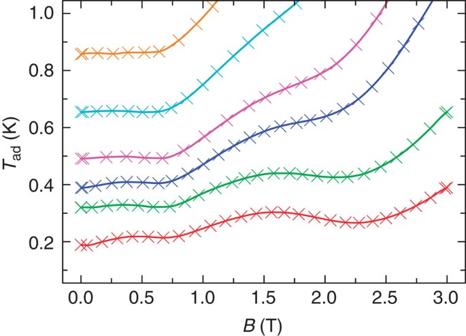Figure 4: Experimental temperature evolution of Gd7on applied field changes. The different curves (which correspond to isentropes) are for different initial temperature and applied field conditionsT0andB0, respectively; solid lines are guides to the eye. The magnetic entropy values areS/R=1.6, 2.9, 3.5, 4.4, 5.9 and 7.6, from bottom to top, respectively. Data are shown for the sub-Kelvin temperature regime (seeSupplementary Fig. 4for a wider temperature range). Figure 4: Experimental temperature evolution of Gd 7 on applied field changes. The different curves (which correspond to isentropes) are for different initial temperature and applied field conditions T 0 and B 0 , respectively; solid lines are guides to the eye. The magnetic entropy values are S / R =1.6, 2.9, 3.5, 4.4, 5.9 and 7.6, from bottom to top, respectively. Data are shown for the sub-Kelvin temperature regime (see Supplementary Fig. 4 for a wider temperature range). Full size image On demagnetization from B 0 =3 T, a minimum (at 2.2 T) is found in the isentropes, that is, the sample cools rapidly (large positive slope) then heats (negative slope), strongly reminiscent of the behaviour observed recently for a 1D AF chain at a quantum critical point [3] . On decreasing the field further, the T ( B ) curves go through a second minimum (at ~0.7 T). As far as we are aware, such multiple peak behaviour has not been observed previously. However, secondary minima have been predicted theoretically for ideal frustrated 2D lattices as a function of decreasing size [5] , [7] , and also for very high-symmetry (cuboctahedral, icosidodecahedral) frustrated clusters [10] , [11] , [12] , [13] , that is, they arise as a function of finite-size effects. Comparison with calculated results We have calculated theoretical isentropes from the entropy function S ( T , B ) based on the parameters from spin Hamiltonian (2) (see Fig. 5c ). We have done this for the experimental entropies that belong to the isentropes shown in Fig. 4 to allow a direct comparison, and for a lower entropy to emphasize the shape of the isentropes. The agreement with the experimental curves is remarkable, showing the double minimum in T ( B ) and consequent multiple cooling regimes. The agreement becomes poorer for the lowest temperatures and small fields because the aforementioned dipolar interactions become relevant. The latter, which are not included in our model, ultimately limit the base temperature reached by adiabatic demagnetization. Analysing the Zeeman diagram is difficult because of the massive (8 7 ) number of levels; in Fig. 5a , we plot the excitation energies ( E *= E i − E 0 , where E i and E 0 are the energies of the ith and ground Zeeman states, respectively, at that field) to make the changes in density of states in certain field ranges more visible. The zero-temperature saturation field is ~2.9 T (that is, above which the ground state is singly degenerate and the magnetic entropy is nil; Fig. 5b ). Below this saturation field, there is a high degeneracy of low-lying states (high entropy), hence rapid magnetic cooling is observed on demagnetizing towards 2.5 T (positive slope isentrope; Fig. 5c ). Between about 2.2 and 1.4 T, the density of states is much lower ( Fig. 5a ), giving a plateau in the zero-temperature magnetization curve ( Fig. 5b ), hence demagnetizing into this region decreases the entropy and leads to heating (negative slope isentrope; Fig. 5c ). Below 1.4 T, the density of states increases again, and we are back in a region of cooling. 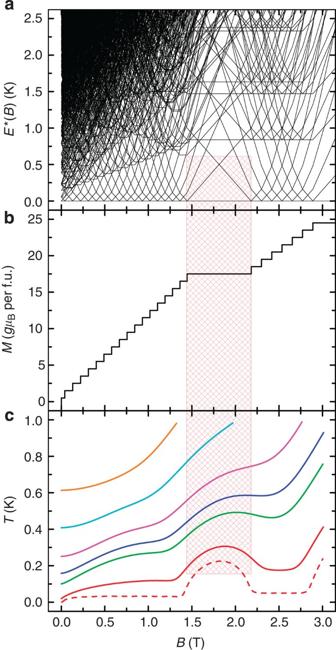Figure 5: Calculated level structure and isentropes for Gd7. (a) Zeeman diagram for Gd7calculated from spin Hamiltonian (2), shown as excitation energies (E*=Ei−E0; whereEiandE0are the energies of the ith and ground Zeeman states, respectively, at a givenB) as a function of applied field, highlighting the varying low-lying density of states. (b) Calculated zero-KelvinM(B) curve. The plateau atM=35/2gμBbetweenB=1.4 and 2.2 T coincides with the region of low density of states ina; saturation (at 49/2gμB) is achieved atB=2.9 T. (c) Theoretically calculated isentropes for magnetic entropy valuesS/R=1.0, 1.6, 2.9, 3.5, 4.4, 5.9 and 7.6, from bottom to top, respectively. The solid lines are those isentropes that match the experimental entropies inFig. 4and can be compared with these directly. The red dashed curve shows a further low-entropy isentrope, lower than those experimentally accessible. The shaded red box highlights the magnetic field region giving the low density of states, the magnetization plateau and the maximum in the isentropes. Figure 5: Calculated level structure and isentropes for Gd 7 . ( a ) Zeeman diagram for Gd 7 calculated from spin Hamiltonian (2), shown as excitation energies ( E *= E i − E 0 ; where E i and E 0 are the energies of the ith and ground Zeeman states, respectively, at a given B ) as a function of applied field, highlighting the varying low-lying density of states. ( b ) Calculated zero-Kelvin M ( B ) curve. The plateau at M =35/2 gμ B between B =1.4 and 2.2 T coincides with the region of low density of states in a ; saturation (at 49/2 gμ B ) is achieved at B =2.9 T. ( c ) Theoretically calculated isentropes for magnetic entropy values S / R =1.0, 1.6, 2.9, 3.5, 4.4, 5.9 and 7.6, from bottom to top, respectively. The solid lines are those isentropes that match the experimental entropies in Fig. 4 and can be compared with these directly. The red dashed curve shows a further low-entropy isentrope, lower than those experimentally accessible. The shaded red box highlights the magnetic field region giving the low density of states, the magnetization plateau and the maximum in the isentropes. Full size image Several frustrated antiferromagnets, including 2D kagome and triangular lattices and certain 0D polytopes, have been predicted to show plateaus in their zero-temperature magnetization curves together with regions of lower densities of states [5] , [7] , [10] , [11] , [12] , [13] . The uneven distributions of intervals between ground-state level crossings is a clear signature of frustration [13] , and is the reason for the peaks observed in the isentrope distribution. This frustration arises because J 1 ≈ J 2 , and test calculations show that the isentrope peaks are quickly destroyed by smaller values of J 2 / J 1 (hence, weakening the frustration; Supplementary Fig. 5 ). Insight into the microscopic origin of the zero-Kelvin magnetization plateau in Gd 7 is gained from evaluating the ground-state nearest-neighbour spin–spin correlation functions as a function of the applied field ( Fig. 6 ), evaluated by numerical differentiation of the ground-state energy with respect to J 1 ( S 12 ) or J 2 ( S 17 ). Calculation from the ground-state eigenfunctions is prohibitive given the enormous Hilbert space. The S 12 function, that is, for neighbouring spins on the hexagon, grows from a fully antiparallel alignment (maximum negative S 12 ) at B =0 to a saturated parallel alignment (maximum positive S 12 ) at B =1.4 T. The S 17 function, that is, for a spin on the hexagon correlated with the central spin, starts at a small negative value and becomes more negative with increasing B , reaching a fully antiparallel alignment at B =1.4 T. S 17 is then constant until B =2.2 T after which it increases, reaching full parallel alignment at B =2.9 T (and saturation of the magnetization at 49/2 gμ B per molecule). Hence, the magnetization plateau between 1.4 and 2.2 T corresponds to a region of stability for the spin configuration with all the spins on the hexagon fully aligned parallel with each other but fully antiparallel to the central spin, consistent with the calculated plateau magnetization of 35/2 gμ B per molecule ( Fig. 5b ). In fact, the Gd 7 structural motif is one of the smallest fragments of the triangular AF net that would be predicted to show such effects. For example, the smallest possible frustrated fragment—an equilateral triangle—has no such ‘meta-stable’ intermediate spin configuration, hence no magnetization plateau and a much simpler isentrope structure ( Supplementary Fig. 6 ). 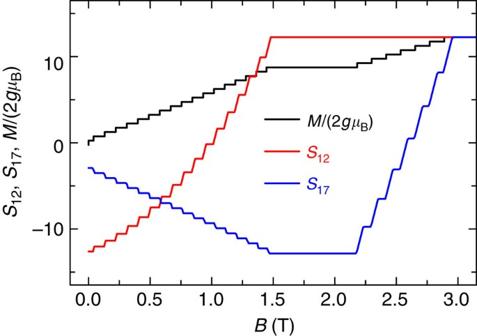Figure 6: Ground-state nearest-neighbour spin correlation functions. The spin functionsare calculated as a function of applied magnetic field.S12measures the correlation of neighbouring spins on the hexagon, whileS17those of a spin on the hexagon and the central spin. |Sij|=49/4 corresponds to full (anti)parallel alignment. The zero-temperatureM(B) curve (scaled by 2gμB) is included to highlight the coincidence of the magnetization plateau with the spin configuration corresponding to the full antiparallel alignment of the central spin with all the other spins. Figure 6: Ground-state nearest-neighbour spin correlation functions. The spin functions are calculated as a function of applied magnetic field. S 12 measures the correlation of neighbouring spins on the hexagon, while S 17 those of a spin on the hexagon and the central spin. | S ij |=49/4 corresponds to full (anti)parallel alignment. The zero-temperature M ( B ) curve (scaled by 2 gμ B ) is included to highlight the coincidence of the magnetization plateau with the spin configuration corresponding to the full antiparallel alignment of the central spin with all the other spins. Full size image Many molecular nanomagnets have now been proposed for low-temperature magnetic refrigeration (see, for example, refs 17 , 19 , 20 , 21 , 22 , 23 , 24 , 25 , 26 ), even in principle to the single-molecule level [27] , due to the high magnetic degeneracies that can be built in by appropriate choice of metal ion and a favourable exchange coupling scheme. Almost all these studies have relied on indirect MCE measurements from magnetization or heat capacity data, which are analysed to predict some maximum magnetic entropy change for a maximum field change (typically 0–5 T on a conventional SQUID magnetometer) and certain initial temperature. Such indirect analyses can give impressive headline figures but ignore the details of the exchange coupling (other than, for example, being ‘weak’, hence giving large quasi-degeneracies in zero field). Hence, they are blind to the structure and true beauty of the isentropes that are a function of the exchange couplings. Here we have revealed the richness of the isentropes in Gd 7 via direct MCE studies, including the first experimental achievement of sub-Kelvin cooling with a molecular nanomagnet, with experimental and theoretical results in excellent agreement. Our results show that it is possible to design the cooling power of molecular materials by choosing an appropriate topology of magnetic couplings between the interacting spins, hence exploiting the great control of the latter given by molecular coordination chemistry. The enhanced MCE we observe in certain regions of the T – B plane for Gd 7 also confirms long-standing predictions about unusually large cooling rates in frustrated spin 0D polytopes as well as low-dimensional extended spin lattices [5] , [6] , [7] , [8] , [9] , [10] , [11] , [12] , [13] . Indeed, the Gd 7 molecule is a cutout of the triangular AF lattice, with imposed geometric spin frustration giving exact or near degeneracies at certain applied magnetic fields, and serves as a finite-size realization of these predictions. Such finite systems are useful in their own right, as demonstrated here, but also enable exact numerical analysis, hence giving insight into the behaviour of infinitely extended systems. If bigger molecular fragments of the triangular AF net could be prepared (such molecules are known for some d-block ions, see refs 28 , 29 ), this would allow fascinating insight into the transition from discrete to bulk behaviour in frustrated systems. Materials [Gd 7 (OH) 6 (thmeH 2 ) 5 (thmeH)(tpa) 6 (MeCN) 2 ](NO 3 ) 2 (‘Gd 7 ’) was prepared as reported previously [14] . Its diamagnetic and isostructural analogue [Y 7 (OH) 6 (thmeH 2 ) 5 (thmeH)(tpa) 6 (MeCN) 2 ](NO 3 ) 2 (‘Y 7 ’) was prepared by an identical method but with substitution of the appropriate metal precursor. Solvothermal reaction of Y(NO 3 ) 3 ·6H 2 O (0.085 g, 0.22 mmol) with H 3 thme (0.11 mmol), Htpa (0.11 mmol) and NEt 3 (0.165 mmol) in MeCN (8 ml) at 100 °C for 12 h, followed by slow cooling (0.05 °C min −1 ) to room temperature, gave colourless crystals of the product in ~40% yield. The formulation is confirmed by elemental analysis, powder X-ray diffraction ( Supplementary Fig. 7 ) and a single-crystal unit cell determination, which show that Y 7 is isostructural with Gd 7 . Elemental analysis (%) for Y 7 C 154 H 164 N 4 O 42 (found:calculated): C 53.26:54.96; H 4.45:4.91; N 1.74:1.66. Measurements Magnetization measurements down to 2 K and heat capacity measurements using the relaxation method down to 0.3 K were carried out on powdered crystalline samples by means of commercial setups for the 0–9 T magnetic field range. Susceptibility measurements were extended down to 0.1 K with a homemade susceptometer, installed in a 3 He- 4 He dilution refrigerator. Direct MCE measurements were performed on a pressed pellet sample mounted on a sapphire plate attached to a Cernox resistance thermometer, attached by wires to a controlled thermal bath. Each MCE measurement started with the sample at zero applied magnetic field and at temperature T 0 , and comprised: (a) gradual application of a magnetic field, up to a maximum B 0 ; (b) relaxation until the sample reached the thermal equilibrium with the bath; (c) gradual demagnetization down to B =0; and (d) relaxation at zero field until the sample reached thermal equilibrium at T 0 . During the whole procedure, the temperature T and applied magnetic field B were recorded continuously. See Supplementary Note 1 for full details. How to cite this article : Sharples, J. W. et al. Quantum signatures of a molecular nanomagnet in direct magnetocaloric measurements. Nat. Commun. 5:5321 doi: 10.1038/ncomms6321 (2014).